Unified metal-free intermolecular Heck-type sulfonylation, cyanation, amination, amidation of alkenes by thianthrenation Direct and site-selective C-H functionalization of alkenes under environmentally benign conditions represents a useful and attractive yet challenging transformation to access value-added molecules. Herein, a unified protocol for a variety of intermolecular Heck-type functionalizations of C sp2 -H bond of alkenes has been developed by thianthrenation. The reaction features metal-free and operationally simple conditions for exclusive cine -selective C-H functionalization of aliphatic and aryl alkenes to forge C-C, C-N, C-P, and C-S bonds at room temperature, providing a general protocol for intermolecular Heck-type reaction of alkenes with nucleophiles (Nu = sulfinates, cyanides, amines, amides). Alkenes undergo cine -sulfonylation, cyanation, amination to afford alkenyl sulfones, alkenyl nitriles and enamines. Alkenes represent one of the most useful functional groups due to their profound potential to a myriad of other functional groups as well their orthogonal reactivity over other polar functional groups [1] , [2] , [3] , [4] . Owing to the abundance, diversity, and easy-availability of alkenes, developing efficient and practical functionalizations of alkenes has been a long-term preoccupation in synthetic chemistry [5] , [6] . Among which, Heck reaction is one of the most straightforward and efficient means to functionalize alkenes [7] , [8] , [9] . Typically, Heck reaction gives access to ipso -substitution of alkenes where a leaving group is bonded to the olefinic carbon atom by nucleophilic species. Comparably, cine -substitution of Heck reaction are less investigated. Over the past decades, transition-metal-catalyzed Heck-type cine -arylation and vinylation of electron-deficient alkenes bearing a leaving group have been developed [10] , [11] , [12] , [13] , [14] , [15] , [16] , [17] , [18] . Straightforward and environmentally benign Heck-type methods that transform alkenes into versatile carbon electrophiles would be highly desirable [19] , [20] . In particular, alkenyl sulfones, alkenyl nitriles, enamines, and enamides are of importance in pharmaceuticals, biochemistry, and materials sciences [21] , [22] , [23] , [24] , providing a straightfoward opportunity in multistep organic synthesis or covalent modification of proteins in drug discovery to couple with different electrophiles. Therefore, direct and regioselective sulfonylation, cyanation, amination, amidation of alkenes would be an enabling synthetic tool to access such privileged structures. To date, metal-free intermolecular Heck-type reaction of alkenes to access alkenyl sulfones [25] , alkenyl nitriles [26] , enamines, and enamides remains underdeveloped [27] , [28] . On the other hand, alkenyl thianthrenium salts [29] , [30] , [31] , [32] , [33] , [34] , [35] , [36] , [37] , [38] , [39] , [40] have been considered as one umpolung strategy of alkenes for further chemical synthesis pioneered by Shine [41] , [42] . Recently, Ritter developed the practical and scalable synthesis of alkenyl thianthrenium salts [43] , [44] , creating new opportunities for derivatization of unactivated alkenes [15] , [45] , [46] . In particular, metal-free functionalization of alkenes represent an attractive aspect to functionalize alkenes under mild conditions. In 2021, elegant examples of electrochemical aziridination of alkenes with primary amines have been demonstrated with or without thianthrene [47] , [48] . The generation of dicationic intermediates also offers potential opportunities for ipso - and cine -substitution reactions. In 2022, Shu group developed a unified metal-free intermolecular aziridination and cyclopropanation of alkenes by thianthrenation (Fig. 1b , top) [49] . Sulfonamides, carbamates, amides, primary amines, and methylenes with acidic protons were all successfully employed as nucleophiles. In 2021, Wickens and Shu independently reported the allylic functionalizations of alkenes by thianthrenation to from C–N, C–C, C–O, and C–S bonds in the presence of nucleophiles (Fig. 1b , middle) [50] , [51] . Recently, Soós group developed an ene-type Kornblum-Ganem oxidation of alkenes by thianthrenation to access various α,β-unsaturated carbonyls (Fig. 1b , bottom) [52] . Interestingly, metal-free transformations of alkenes by thianthrenation basically led to bond-formation at ipso -carbon of alkenyl thianthrenium salts. We questioned the possibility of realizing a new bond-formation mode of alkenyl thianthrenium salts to functionalization cine -carbon of alkenes under metal-free conditions [48] . Herein, we report a unified protocol for metal-free cine -functionalizations of alkenes by thianthrenation (Fig. 1c ). The reaction explores the new reactivity of alkenyl thianthrenium salts to form a new chemical bond at cine -position instead of ipso -position of vinyl thianthrenium salts. The mild condition allows for the site-selective C–H functionalization of alkenes to forge C–S, C–N, C–P and C–C bonds with diverse nucleophiles. Fig. 1: Impetus for metal-free functionalizations of alkenes by thianthrenation. a Transition-metal-catalyzed cine -substitution of alkene electrophiles. b Representative metal-free functionalization modes of alkenes by thiathrenation. c Metal-free cine -functionalizations of alkenes by thianthrenation (this work). Full size image 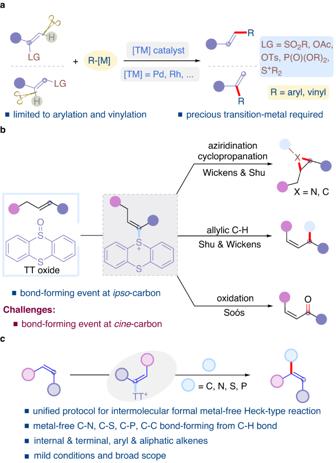Fig. 1: Impetus for metal-free functionalizations of alkenes by thianthrenation. aTransition-metal-catalyzedcine-substitution of alkene electrophiles.bRepresentative metal-free functionalization modes of alkenes by thiathrenation.cMetal-freecine-functionalizations of alkenes by thianthrenation (this work). Optimization of the reaction conditions We started the investigation using sodium methanesulfinate ( 1a ) and 4-phenylbut-1-enylthianthrenium salt ( 2a ) as model substrates to evaluate the reaction conditions (Table 1 ). To our delight, cine -sulfonation of the C = C bond of the vinyl thianthrenium salt was exclusively formed, without the formation of formal allylic C-H sulfonation byproduct ( 3a’ ) as previously reported. After evaluation of the reaction parameters, we define the reaction in DCE (0.1 M) at room temperature without any additive as standard conditions, providing the desired product (3-(methylsulfonyl)but-3-en-1-yl)benzene 3a in 83% isolated yield (Table 1 , entry 1). The use of other solvents instead of DCE could also mediate the desired transformation, albeit giving 3a in lower yields (Table 1 , entries 2–9). Table 1 Condition evaluation for the cine -sulfonation. a Full size table Scope of the reaction With the optimized conditions in hand, the scope of alkenes and sodium sulfinates is examined and the results are summarized in Fig. 2 . First, the scope of alkenes was evaluated. A wide range of alkenes with diverse electronic and steric properties are suitable for this reaction, allowing the corresponding cine -sulfonylation of alkenes by thianthrenation with sodium methanesulfinate in good yields ( 3a - 3z ). Aliphatic terminal alkene-based thianthrenium salts are all compatible in this reaction, producing alkenyl sulfones in 52–88% yields ( 3a - 3m ). Alkenes with pendant amides, bromides, esters were compatible in the reaction, giving the corresponding cine -substitution products ( 3c, 3d, 3g - 3i ) in 69–88% yields. It is noteworthy that amides with free N–H, free alcohols, and alkenes were all compatible in the reaction to furnish the desired alkenyl sulfones ( 3h, 3j , and 3k ) in 70–75% yields, leaving chemical space for further elaboration. In addition, α-branched aliphatic alkene-based thianthrenium salts are also good substrates in the reaction, giving corresponding cine -sulfonylation products in 81% and 85% yields ( 3l and 3m ). Moreover, styrenes could be efficiently involved in the cine -substitution process by thianthrenation, giving the desired sulfones in 61–92% yields ( 3n - 3s ). In addition, cyclic alkenes were easily converted to alkenylsulfones in 59–89% yields ( 3t - 3w ) under the reaction conditions. Notably, gaseous alkenes, such as ethylene and propene, could be successfully involved in this cine -substitution process by thianthrenation, giving 3e, 3x and 3y in 52–88% yields. Lithocholic acid drived alkene with molecular complexity underwent cine -substitution process smoothly, giving the desired product ( 3z ) in 70% yield. Fig. 2: Scope of cine -sulfonylation of alkenes by thianthrenation. Standard conditions, see Table 1 for details. Isolated yield is shown. a Reaction was run for 24 h. b Reaction was conducted at 50 o C. c Reaction was run at 50 o C for 36 h. d Reaction was conducted on 4.0 mmol scale. Full size image Next, the scope of sulfinates was tested. para -Substituted aryl sulfinates with electron-donating ( 4a - 4d ) or electron-withdrawing ( 4e - 4i ) groups were all well-tolerated in this reaction, giving corresponding cine -sulfonylation products in good yields (61–96%). Moreover, meta - and ortho -substituted aryl sulfinates were also good substrates for this reaction to give the desired products ( 4j and 4k ) in 76% and 60% yields, respectively. Fused aryl and heteroaryl sulfinates underwent cine -substitution to give the desired products ( 4l and 4m ) in 79% and 89% yields. Vinyl sulfinate proceeded smoothly to give the corresponding alkenyl sulfone 4n in 84% yield. Notably, allylic, acyclic and cyclic alkyl sulfinates were compatible in this metal-free cine -substitution process and afforded the corresponding sulfones in 65-90% yields ( 4o - 4q ). It is noteworthy that bulky sulfinates smoothyl underwent cine -substitution of C-H bond by thianthrenation to give the corresponding alkenyl sulfones in 75% and 86% yields ( 4r and 4s ). In addition, the structure of the alkenyl sulfones was unambiguously confirmed by X-ray diffraction of 4k . The reaction could be scaled up to 4.0 mmol to afford 4a in 84% yield (1.16 g), rendering the reaction useful for large-scale synthesis. Furthermore, the protocol for cine -functionalizations of alkenes by thianthrenation was further applied to cine -cyanation, cine -amination, and cine -amidation to forge C-C bonds and C-N bonds from C-H bonds (Fig. 3 ). With slight modification of the solvent and base, cine -cyanation was achieved with zinc cyanide in the presence of KF (3.0 equiv) in CH 3 CN (0.1 M) at room temperature, delivering the desired 2-methylene-4-phenylbutanenitrile ( 5a ) in 70% isolated yield (Supplementary Tables 2 and 3 ) (for details see Supplementary Information) [48] . Then, the scope of cine -cyanation was evaluated. α-Branched terminal alkene derived thianthrenium salt is compatible with this cine -cyanation, delivering the corresponding cine -substitution product ( 5b ) in 53% yield. Additionally, aliphatic alkenes tethered with esters, amides, alcohols were all compatible in this reaction, affording the desired acrylonitriles in 65-77% yields ( 5c - 5e ). Moreover, alkenes with bromides and alkenes were successfully transformed to the cine -cyanation products in 84% and 47% yields ( 5f and 5g ). Notably, cyclic and acyclic internal aliphatic alkenes derived thianthrenium salts were amenable to this cine -cyanation, affording diverse acrylonitriles in 76% and 46% yields ( 5h and 5i ). Interestingly, styrenes also worked well for this cine -cyanation to afford 5j in 70% yield. Fig. 3: Scope of the cine -cyanation, cine -amination and cine -amidation of alkenes by thianthrenation. The reaction was carried out using 1 (0.15 mmol), 2 (0.10 mmol), KF (3.0 equiv) in CH 3 CN (0.1 M) at room temperature for 10 h unless otherwise stated. Isolated yield is shown. a The reaction was conducted at 50 o C. b The reaction was conducted at 50 o C for 24 h. c The reaction was conducted using K 2 CO 3 (1.0 equiv). rr = ratio of regioisomers. d The reaction was conducted on 5.0 mmol scale using K 2 CO 3 (1.0 equiv). e The reaction was conducted using Cs 2 CO 3 (1.0 equiv). Full size image Impressively, this operationally simple cine -substitution protocol could be successfully applied to cine -amination of C-H bonds using nitrogen nucleophiles (Fig. 3 ). The reaction of 2q with indole in the presence of K 2 CO 3 (1.0 equiv) in CH 3 CN (0.1 M) at room temperature afforded the selective cine -substitution at nitrogen product 1-(1-(4-fluorophenyl)vinyl)-1 H -indole 6a in 82% isolated yield (Supplementary Tables 4 and 5 ) (for details see Supplementary Information). Ketone-, aldehyde-, and bromo-substituted indoles were well-tolerated under this cine -amination conditions, delivering the corresponding N -vinyl indoles ( 6b - 6d ) in 76 − 81% yields. Additionally, carbazole and imidazole were all excellent substrates for this cine -substitution, yielding the desired N -vinyl carbazole ( 6e ) and imidazole ( 6f ) in 81% and 84% yields. Moreover, sulfonamides and amides were smoothly transformed into corresponding N -vinyl amides in 64% and 80% yields ( 6g and 6h ). Furthermore, pyrazoles and 1,2,4-triazoles were remarkable substrates for this cine -substitution reaction, producing the desired N -vinyl pyrazole ( 6i ) and triazole ( 6j ) in 66% and 70% yields. 1,2,3-Triazoles were also compatible in the reaction, delivering a mixture of 6k and 6k’ in 36% and 28% yields. Moreover, a variety of alkenes worked well the C-N bond-forming process from cine -C-H bond of alkenes by thianthrenation. Chloro-, bromo-substituted styrenes and internal styrenes were compatible with this cine -substitution reaction, generating cine -amination products ( 6l - 6n ) in 78-82% yields. Linear and α-branched aliphatic alkenes derived thianthrenium salts were all tolerated under the cine -amination conditions, delivering corresponding enamines ( 6o and 6p ) in 60% and 74% yields. Isolated diene selectively underwent thianthrenation and sequential cine -amination on one alkene, giving corresponding product 6q in 65% yield. Unsymmetrical alkenes could be involved in the regioselective thianthrenation and sequential cine -amination to yield 6r in 73% yield with >15:1 rr. Cyclic alkenes with different ring size could be involved to this cine -substitution with imidazole to furnish enamines ( 6s and 6t ) in 57% yield. Additionally, drug molecules have been derivatized. Metaxalone, and lansoprazole underwent selective cine -amination reaction of the C-H bond of alkenes with amides and benzoimidazoles to give N -acyl and N -aryl enamines ( 6u and 6v ) in 82% and 70% yields, respectively. Interestingly, melatonin underwent chemoselective N -vinylation with of indoles instead of the amides at cine -position of alkenes to give N -aryl enamine derivative ( 6w ) in 75% yield under standard conditions. Additionally, cine -phosphonylation product 7a was got in 69% yield from phosphoryl nucleophile and alkenylthianthrenium salt. Mechanistic study To enhance the practicality of this operationally simple protocol, a one-pot procedure was evaluated for cine -sulfonylation and amination (Fig. 4a ). The one pot thianthrenation of 4-phenyl-1-butene using thianthrene S -oxide, followed by the reaction of sodium methanesulfinate or imidazole under corresponding conditions were conducted, affording the desired cine -substituted products in comparable yields ( 3a , 71%) or ( 6o , 65%) without any intermediate purification. Furthermore, the reactions of 1a and 2a in the presence of 2 equiv of radical scavenger (TEMPO or BHT) were carried out under otherwise identical to standard conditions, providing the desired alkenyl sulfone 3a in 72% and 83% yields (Fig. 4b ). The result that the presence of TEMPO or BHT did not decrease the efficiency of this reaction, excluding the radical pathway of this cine -substitution reaction. To further detect the mechanism of this cine -substitution, the preformed alkyl thianthrenium salts ( 8a and 8b ) were subjected to nucleophiles under standard conditions (Fig. 4c ). Corresponding alkenyl sulfone 3a and alkenyl amine 6o were obtained in 63% and 57% yield, suggesting the primary alkyl thianthrenium salts may serve as the intermediate for the selective cine -substitution process. Additionally, the reaction of 1aa and deuterated alkenyl thianthrenium salt 2cc was conducted under standard conditions, affording the desired cine -amination product 8c in 65% yield. Interestingly, partial deuterium scrambling was observed (Fig. 4d ), supporting the proton exchange of β-position of alkenyl thianthrenium salt with surroundings and protonation of α-position of alkenyl thianthrenium. Fig. 4: One-pot cine -functionalizations of alkenes and mechanistic investigations. a One-pot reactions for cine -substitution of alkenes. b Probe radical nature of the reaction. c Assign reaction intermediates. d Reaction with deuterated vinyl thianthrenium salt. Full size image Based on the mechanistic experiments and literature [48] , [49] , [50] , [51] , [52] , a plausible mechanism of the metal-free cine -substitution of alkenyl thianthrenium salts is proposed and depicted in Fig. 5 . First, the zwitterionic alkyl thianthrenium salt intermediate M1 could be formed by intermolecular addition of nucleophiles on distal position of alkenes to forge C-S/C-C/C-N/C-P bonds. After protonation of M1 to form a more stable intermediate M2, M2 underwent deprotonation on cine -site yield the zwitterion M3 . M3 could undergo intramolecular elimination to afford alkenyl sulfones, acrylonitriles, enamines, and enamides by releasing thianthrene. Fig. 5: Proposed mechanism of the reaction. The plausible mechanism for metal-free cine -functionalization of alkenes by thianthrenation. 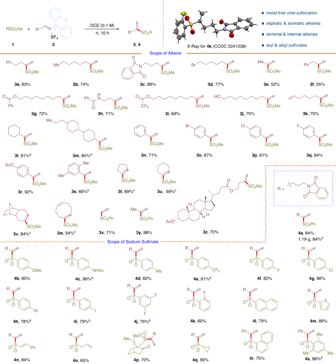Fig. 2: Scope ofcine-sulfonylation of alkenes by thianthrenation. Standard conditions, see Table1for details. Isolated yield is shown.aReaction was run for 24 h.bReaction was conducted at 50oC.cReaction was run at 50oC for 36 h.dReaction was conducted on 4.0 mmol scale. Full size image In conclusion, a unified metal-free protocol for diverse intermolecular cine -functionalizations of the C–H bond of alkenes by thianthrenation has been achieved. The reaction features metal-free C–H functionalizations of alkenes under mild conditions to forge C–S, C–C, C–N, and C–P bonds from C–H bonds via cine -sulfonylation, cine -cyanation, cine -amination, cine -amidation, and cine -phosphonylation. The reaction represents new metal-free reaction mode to functionalize cine -carbon of alkenyl thianthrenium salts, which is complementary to previous functionalization at ipso -carbon. Mechanistic investigations revealed the reaction undergo site-selective nucleophilic addition followed by regioselective elimination to afford the formal Heck reaction of alkenes, affording synthetic useful synthons which are difficult to access from readily accessible starting materials. General procedure A for intermolecular Heck-type sulfonylation of alkenes by thianthrenation Sodium sulfinate (0.15 mmol) and vinyl thianthrenium salt (0.1 mmol) were placed in a 10.0 mL Schlenk tube which equipped with a magnetic stir bar. After back-filled with nitrogen (this process was repeated three times), DCE (1.0 mL) was added. The vial was sealed and at room temperature (for the large hindrance substrates its require at 50 °C) with stirring until TLC indicated the complete consumption of thianthrene (typically 10 h or 36 h). The reaction mixture was evaporated and purified directly by column chromatography to afford the product. General procedure B for intermolecular Heck-type cyanation of alkenes by thianthrenation Zn(CN) 2 (17.6 mg), KF (17.4 mg) and vinyl thianthrenium salt (0.1 mmol) were placed in a 10.0 mL Schlenk tube which equipped with a magnetic stir bar. After back-filled with nitrogen (this process was repeated three times), CH 3 CN (1.0 mL) was added. The vial was sealed and at room temperature (for the large hindrance substrates it require at 50 °C) with stirring until TLC indicated the complete consumption of thianthrene (typically 10 h or 24 h). The reaction mixture was evaporated and purified directly by column chromatography to afford the product. General procedure C for intermolecular Heck-type amination and amidation of styrenes by thianthrenation Nucleophile (0.15 mmol), K 2 CO 3 (13.8 mg) and vinyl thianthrenium salt (0.1 mmol) were placed in a 10.0 mL Schlenk tube which equipped with a magnetic stir bar. After back-filled with nitrogen (this process was repeated three times), CH 3 CN (1.0 mL) was added. The vial was sealed and at room temperature with stirring until TLC indicated the complete consumption of thianthrene (typically 10 h). 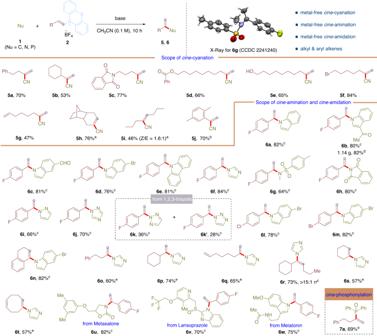Fig. 3: Scope of thecine-cyanation,cine-amination andcine-amidation of alkenes by thianthrenation. The reaction was carried out using1(0.15 mmol),2(0.10 mmol), KF (3.0 equiv) in CH3CN (0.1 M) at room temperature for 10 h unless otherwise stated. Isolated yield is shown.aThe reaction was conducted at 50oC.bThe reaction was conducted at 50oC for 24 h.cThe reaction was conducted using K2CO3(1.0 equiv). rr = ratio of regioisomers.dThe reaction was conducted on 5.0 mmol scale using K2CO3(1.0 equiv).eThe reaction was conducted using Cs2CO3(1.0 equiv). The reaction mixture was evaporated and purified directly by column chromatography to afford the product. 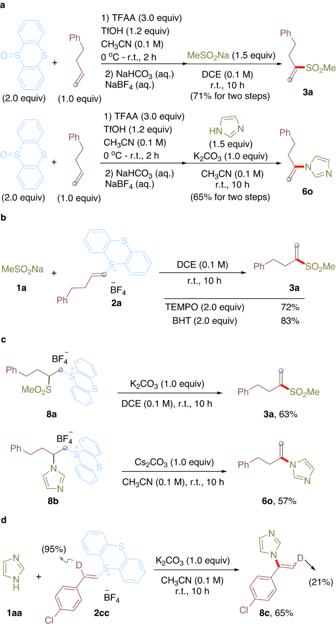Fig. 4: One-potcine-functionalizations of alkenes and mechanistic investigations. aOne-pot reactions forcine-substitution of alkenes.bProbe radical nature of the reaction.cAssign reaction intermediates.dReaction with deuterated vinyl thianthrenium salt. 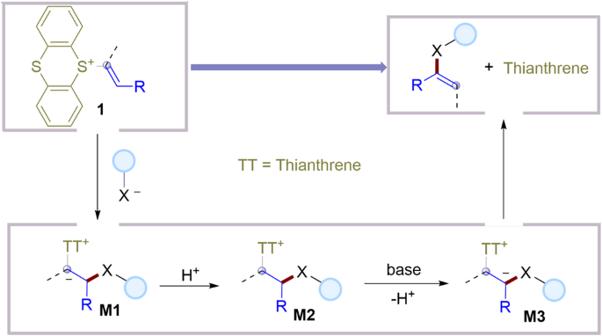Fig. 5: Proposed mechanism of the reaction. The plausible mechanism for metal-freecine-functionalization of alkenes by thianthrenation. General procedure D for intermolecular Heck-type amination and amidation of aliphatic alkenes by thianthrenation Nucleophile (0.15 mmol), Cs 2 CO 3 (32.6 mg) and vinyl thianthrenium salt (0.1 mmol) were placed in a 10.0 mL Schlenk tube which equipped with a magnetic stir bar. After back-filled with nitrogen (this process was repeated three times), CH 3 CN (1.0 mL) was added. The vial was sealed and at room temperature with stirring until TLC indicated the complete consumption of thianthrene (typically 10 h). The reaction mixture was evaporated and purified directly by column chromatography to afford the product.